Biologically enhanced cathode design for improved capacity and cycle life for lithium-oxygen batteries Lithium-oxygen batteries have a great potential to enhance the gravimetric energy density of fully packaged batteries by two to three times that of lithium ion cells. Recent studies have focused on finding stable electrolytes to address poor cycling capability and improve practical limitations of current lithium-oxygen batteries. In this study, the catalyst electrode, where discharge products are deposited and decomposed, was investigated as it has a critical role in the operation of rechargeable lithium-oxygen batteries. Here we report the electrode design principle to improve specific capacity and cycling performance of lithium-oxygen batteries by utilizing high-efficiency nanocatalysts assembled by M13 virus with earth-abundant elements such as manganese oxides. By incorporating only 3–5 wt% of palladium nanoparticles in the electrode, this hybrid nanocatalyst achieves 13,350 mAh g −1 c (7,340 mAh g −1 c+catalyst ) of specific capacity at 0.4 A g −1 c and a stable cycle life up to 50 cycles (4,000 mAh g −1 c , 400 mAh g −1 c+catalyst ) at 1 A g −1 c . Rechargeable Li-O 2 batteries operate through the reversible reaction between lithium ions and oxygen molecules [1] , [2] , [3] . When Li-O 2 batteries discharge in non-aqueous electrolytes, Li + reacts with reduced oxygen (oxygen reduction reaction; ORR) yielding the reaction product, mainly Li 2 O 2 that is deposited on the catalyst electrode at a thermodynamic voltage of 2.96 V (versus Li/Li + ) [4] , [5] , [6] . On charging, the electrical energy is stored by decomposing Li 2 O 2 back into Li + and O 2 (oxygen evolution reaction; OER). To promote these ORR and OER for Li-O 2 batteries, several materials have been investigated as catalyst electrodes, such as noble metals (for example, Au, Pt, Ru and Pd) [7] , [8] , [9] , transition metal oxides (for example, α-MnO 2 (ref. 10 ), Co 3 O 4 (ref. 11 ), MnCo 2 O 4 (ref. 12 ), RuO 2 (ref. 13 )) and carbon-based materials (for example, graphene [14] , [15] , carbon fibre [16] and doped carbon nanotube [17] ). However, these materials suffer either from high material costs, low conductivities or side reactions with electrolytes, which limits their use as high-performance Li-O 2 battery electrodes. Although these difficulties restrain the capability of Li-O 2 batteries, the rational design and selection of electrode materials may fully deliver these battery chemistries to a high gravimetric energy storage system. To enhance structural functionality, organisms in nature form skeletal tissues from soft to hard through the interactions between nucleating protein matrices and inorganic ions [18] , [19] , [20] . Inspired by these biominerals, researchers have fabricated novel nanoarchitectures using peptides or proteins as scaffolds applied in various functional structures [21] . For example, numerous types of platforms such as synthetic peptide nanofibers [22] , nanorings [23] and ferritin cages [24] provide simple and uniform ways to synthesize interesting materials at the nanoscale. In electrochemical energy storage devices, nanostructured materials enhance Li ion batteries by shortening the diffusion length of Li ions [25] , [26] , [27] and benefit capacitors by providing electrodes with large surface areas [28] , [29] . For Li-O 2 batteries, as the oxygen is in principle derived from the air, both oxygen flow into electrodes and the high efficiency to promote discharge/charge reactions are additional important factors [30] . Constructing a new catalyst that combines porous nanostructures and high catalytic activity would allow us to harness the advantages of Li-O 2 batteries for practical applications, such as long-range electric vehicles. Here we built the catalyst structures to achieve high Li-O 2 battery performances by forming a nanocomposite of biotemplated manganese oxide nanowires (bio MO nanowires) with incorporation of a small weight percent (3 wt%) of Pd nanoparticles ( Fig. 1 ). We believe this is the first bio-directed synthetic method demonstrated for Li-O 2 battery applications. 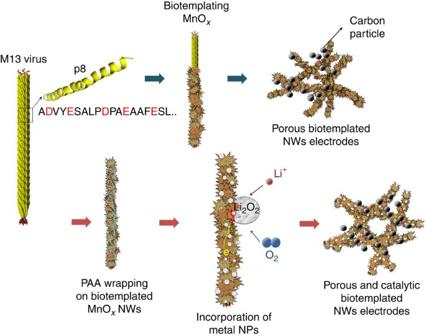Figure 1: Schematic of a nanocomposite structure Synthesis step of the metal nanoparticle/M13 virus-templated manganese oxide nanowires (bio MO nanowires) and the operational reaction inside Li-O2battery cells. Figure 1: Schematic of a nanocomposite structure Synthesis step of the metal nanoparticle/M13 virus-templated manganese oxide nanowires (bio MO nanowires) and the operational reaction inside Li-O 2 battery cells. Full size image M13 virus-mediated synthesis of manganese oxide nanowires Bio MO nanowires with spherulitic surface morphology were synthesized through a facile and moderate chemical reaction by utilizing the biomolecule, M13 virus. M13 viruses have been used as versatile templates for high aspect ratio nanowire synthesis (for example, semiconductors [31] , metal oxides [32] , [33] , [34] ) under environmentally benign conditions. Among the five different types of capsid proteins on this virus template, p8 is a major coat protein with 2,700 copies surrounding the single-stranded DNA. In addition to the material specificity of these surface proteins (p8 or five copies of minor proteins existing at one end of virus particle, p3), electrostatic interactions between the opposite charge of precursor ions and functional groups of p8 coat protein broaden the template functionality. In this work, the virus clone with the p8 peptide sequences ADVYESALPDPAEAAFE (named FC#2) [35] was used because it has two additional negative functional groups (-COOH from glutamic acid on 13th and 17th) than M13KE (New England Biolabs) under basic conditions. Using this clone, bio MO nanowires were synthesized by first binding Mn 2+ ions to the FC#2 virus p8 proteins followed by reacting with KMnO 4 at room temperature. From this simple aqueous biotemplating reaction, homogeneous bio MO nanowires with high aspect ratio (~80 nm in diameter and ~1 μm in length) were obtained. These nanowires showed spherulitic surface morphology (transmission electron microscopy (TEM) image in Fig. 2a,b and Supplementary Fig. S1a ). Although the flower-like spheres of MO were previously synthesized [36] , [37] , the nucleation of MO along the virus particle developed this spherulitic surface of materials into higher-dimensional nanowires. Thus, the hierarchical nanostructures of these bio MO nanowires are expected to be advantageous in Li-O 2 battery performances. Although previous studies utilized smooth surface MO nanowires for Li-O 2 battery electrodes [10] , [38] , the rough surface of these bio MO nanowires can provide large catalytic area as well as enough storage space for discharge products. To the best of our knowledge, this is the first report of M13 virus-directed synthesis of manganese oxide nanowires, which is applicable not only to Li-O 2 battery electrodes but also to various applications such as electrochemical capacitors [39] , Li ion battery electrodes [40] and water purifications [41] . 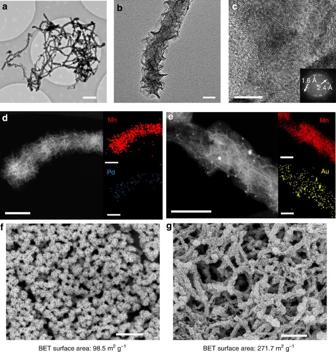Figure 2: Electron microscope images of catalyst materials. TEM images of M13 virus-templated MO nanowires (a) at low magnitude (scale bar, 500 nm), (b) zoomed at the end of an individual bio MO nanowire (scale bar, 50 nm) and (c) HRTEM image showing amorphous phase mixed with crystalline phase (scale bar, 5 nm, inset: the fast Fourier transform (FFT) pattern with two major rings matching to the atomic planes with the spacing of 2.4 and 1.6 Å, respectively). The synthetic procedure of bio MO nanowires was easily reproducible. We synthesized, characterized and made electrodes from over 30 times independent experiments. (d) STEM image of Pd/bio MO nanowires (left) and the corresponding energy dispersive X-ray (EDX) elemental mapping images of manganese (Mn, red, upper right) and palladium (Pd, blue, lower right; scale bars, 100 nm). (e) STEM image of Au/bio MO nanowires (left) and the corresponding EDX elemental mapping images of manganese (Mn, red, upper right) and gold (Au, yellow, lower right; scale bars, 50 nm). The SEM image and BET surface area of (f) MO nanoparticle showing bulky phase of aggregated particles and (g) homogeneously dispersed bio MO nanowires with larger pores (scale bars, 500 nm). The two BET surface areas are 98.5 (f) and 271.7 m2g−1(g). Figure 2: Electron microscope images of catalyst materials. TEM images of M13 virus-templated MO nanowires ( a ) at low magnitude (scale bar, 500 nm), ( b ) zoomed at the end of an individual bio MO nanowire (scale bar, 50 nm) and ( c ) HRTEM image showing amorphous phase mixed with crystalline phase (scale bar, 5 nm, inset: the fast Fourier transform (FFT) pattern with two major rings matching to the atomic planes with the spacing of 2.4 and 1.6 Å, respectively). The synthetic procedure of bio MO nanowires was easily reproducible. We synthesized, characterized and made electrodes from over 30 times independent experiments. ( d ) STEM image of Pd/bio MO nanowires (left) and the corresponding energy dispersive X-ray (EDX) elemental mapping images of manganese (Mn, red, upper right) and palladium (Pd, blue, lower right; scale bars, 100 nm). ( e ) STEM image of Au/bio MO nanowires (left) and the corresponding EDX elemental mapping images of manganese (Mn, red, upper right) and gold (Au, yellow, lower right; scale bars, 50 nm). The SEM image and BET surface area of ( f ) MO nanoparticle showing bulky phase of aggregated particles and ( g ) homogeneously dispersed bio MO nanowires with larger pores (scale bars, 500 nm). The two BET surface areas are 98.5 ( f ) and 271.7 m 2 g −1 ( g ). Full size image With the aqueous, room temperature approach using M13 virus templates, multivalent (Mn 3+ /Mn 4+ ), birnessite-like MO nanowires were developed. The crystallographic and chemical properties of bio MO nanowires were investigated with X-ray diffraction (XRD), high-resolution TEM (HRTEM), the chemical titration method and X-ray photoelectron spectroscopy (XPS). First, the XRD pattern of virus-templated MO nanowires showed three broad peaks centred at 2 θ of 37°, 53.5° and 65.5° ( Supplementary Fig. S1b ), partially matching to δ-MnO 2 (birnessite, space group C2/m, powder diffraction file number 01-073-2509) XRD pattern. In addition, the surface morphology of bio MO nanowires was similar to that of typical birnessites [42] , as can be seen in the TEM image ( Fig. 2b ). The crystal sizes of bio MO nanowires were 2–5 nm and the coexisting amorphous phase was observed by HRTEM ( Fig. 2c ). The average oxidation state of bio MO nanowires was determined to be 3.51 by chemical titration methods [43] , suggesting a multivalence state (Mn 3+ /Mn 4+ =0.96) of nanowires. This mixed-valence property of MO was also observed from XPS spectra in Supplementary Fig. S2 . We confirmed that the average oxidation state of bio MO nanowires lies between Mn 3+ and Mn 4+ by observing two features: the peak position of Mn 2p 3/2 and the multiplet splitting of Mn 3s. First, the Mn 2p 3/2 peak position of bio MO nanowires (642.1 eV in Supplementary Fig. S2a ) was close to that of MnO 2 (Mn 4+ , 642.2~642.4 eV) as reported in the literature [44] , [45] . However, the width of Mn 3s multiplet splitting (5.2 eV in Supplementary Fig. S2b ) of bio MO nanowires showed a larger separation than that of MnO 2 (4.5~4.7 eV) but close to that of Mn 2 O 3 (5.2~5.4 eV) [44] , [45] . As it is known that the separation between Mn 3s splitting peaks becomes larger as the oxidation state of Mn is lower [46] , the larger separations of Mn 3s splitting compared with Mn 4+ imply the presence of a lower valence state in bio MO nanowires. Nanocompositing ORR catalyst on bio MO nanowires To enhance the ORR activity and surface conductivity of porous bio MO nanowires for Li-O 2 battery electrodes, 1–3 wt% of ORR catalytic metal nanoparticles were homogeneously incorporated onto the surface of the nanowires. It is reported that noble metal nanoparticles (for example, Pd, Pt, Ru and Au) have higher intrinsic ORR activities compared with carbon with 0.1 M lithium perchlorate (LiClO 4 ) in dimethoxyethane (DME) electrolyte [7] . In particular, very recent studies reported a great stability (Au) [47] and high ORR catalytic activity (Pd) [7] in Li-O 2 battery applications. However, those electrodes contained 40–100 wt% of noble metal nanoparticles, making them less practical because of cost-efficiency. Thus, we suggest the composite structure of bio MO nanowires combined with noble metal nanoparticles to decrease the loading of precious metals in cathodes while maximizing the catalytic activity of Li-O 2 batteries. The nanocomposites were designed to nucleate the metal nanoparticle on the surface of the bio MO nanowire templates to maximize the contact with discharge products in Fig. 1 (red lines, right middle). In addition, the homogeneous distribution of ORR metal catalyst along the bio MO nanowires was important in maintaining the porous structure of the electrodes. To facilitate these requirements, poly acrylic acid (PAA) was incorporated around the bio MO nanowires to nucleate the metal nanoparticle. The PAA-wrapped nanowires increased the colloidal stability of the nanowires during the synthesis so that a more homogeneous solution of bio MO nanowires was observed ( Supplementary Fig. S3 ). Control experiment without PAA wrapping resulted in free Pd nanoparticle formation and aggregated MO nanowires as shown in the TEM image ( Supplementary Fig. S4 ). This composite synthesis method was applied to two different ORR metal catalysts, Au or Pd (Au/Pd). To nucleate these metal nanoparticles on PAA-wrapped bio MO nanowires, ethylene glycol was used as a mild and selective reducing agent to react with noble metal precursors (HAuCl 4 and Na 2 PdCl 4 ) slowly, avoiding reactions with virus-templated MO nanowires. This metal nanoparticle incorporation method by stabilizing and trapping precursor ions with PAA is expected to be applicable not only to biotemplated nanowires but also to various nanosized substrates, such as nanofibers. The homogeneous distribution of Au/Pd nanoparticles (with a diameter of 2–6 nm Supplementary Fig. S5 ), was observed by elemental mapping using scanning TEM (STEM) in Fig. 2d,e . The amount of PAA used to form the composite nanostructure was determined with thermogravimetric analysis (TGA) to be 2.5 wt% of the electrode by comparing the weight loss difference between bio MO nanowires and Pd incorporated bio MO nanowires at 500°C ( Supplementary Fig. S6 ) [48] . The amount of Au/Pd nanoparticle incorporated in the bio MO nanowires was measured by inductively coupled plasma atomic emission spectroscopy (ICP-AES) analysis and varied ~1–3 wt% of the total electrode, depending on the metal precursor amount that was added during synthesis. Improved Li-O 2 battery performances with bio MO nanowires The virus-templated MO Li-O 2 battery cathodes showed a 9,196 mAh g −1 c (955 mAh g −1 c+catalyst+Li2O2 ) first discharge capacity with 92.6% of coulombic efficiency at a current density of 0.4 A g −1 c . The electrochemical tests were performed with 0.1 M LiClO 4 /DME electrolyte under 1 atm of oxygen (further details on measurement methods are described in the experimental section). Although ether-based electrolytes may undergo some side reactions during Li-O 2 battery charging [49] , it is one of the most stable electrolytes against the oxygen electrode for Li-O 2 batteries known to date [50] without the reactivity with Li metal like DMSO has. [47] Further control experiments with different electrolytes are included in the Methods section and Supplementary Fig. S7 . For galvanostatic tests, the operating voltage was limited to 2.2–4.15 V (versus Li/Li + ) to minimize possible parasitic reactions. First, the effect of MO electrode structures on Li-O 2 battery performance was studied by varying the architecture from nanoparticles to bio MO nanowires. Under the same synthetic conditions, MO nanoparticles (60 nm diameter) were synthesized without viruses and their morphology was compared with bio MO nanowires with scanning electron microscope (SEM) images ( Fig. 2f,g ). The surface area of both nanoparticles and nanowires was measured by the Brunauer–Emmett–Teller (BET) method giving 98.5 and 271.7 m 2 g −1 , respectively. Bio MO nanowires showed a 40% improvement of Li 2 O 2 storage capability (9,196 mAh g −1 c at 0.4 A g −1 c ) compared with MO nanoparticles (6,545 mAh g −1 c ), as can be seen from the first discharge capacity in Fig. 3a . In addition, the discharge voltage of the bio MO nanowires (~2.68 V) is higher than that of MO nanoparticles (~2.6 V) by ~80 mV and the charge voltage of the bio MO nanowires (~3.65 V) is lower than that of MO nanoparticles (~3.77 V) by ~120 mV. In other words, the bio MO nanowires showed decreased discharge and charge overpotentials compared with the MO nanoparticles. As the oxidation state of both MO nanoparticles and nanowires was determined to be similar by XPS analysis ( Supplementary Fig. S2a,b ), the difference in Li-O 2 battery discharge capacity was mainly attributed to their different surface area [51] and morphologies. As MO nanoparticles agglomerate during the synthesis, the low surface area electrode materials ( Fig. 2f ) limit the surface-mediated reaction so that it results in a poor specific discharge capacity. In our biotemplated system, the high aspect ratio as well as larger surface areas ( Fig. 2g ) formed highly active Li-O 2 battery cathodes where the electrode spaces can be fully utilized while minimizing the effect of discharge product blocking the electrodes. 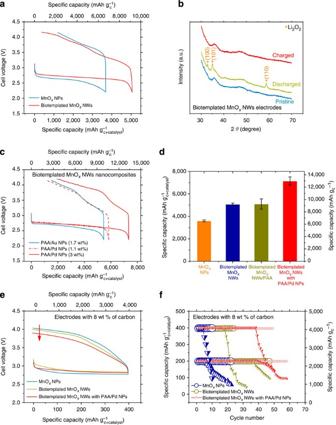Figure 3: The electrochemical performance of Li-O2batteries. (a) The first galvanostatic cycle of MO nanoparticles (blue) and bio MO nanowires (red) at a current density of 0.4 A g−1c(~0.044 mA cm−2) with 0.1 M LiClO4/DME electrolytes under 1 atm oxygen. (b) XRD patterns of bio MO nanowire electrodes at the pristine state (blue), the end of the first full discharge until 2.2 V (dark yellow) and the end of the first full charge until 4.15 V (red) under 0.4 A g−1cof current density. (c) The first galvanostatic cycle of bio MO nanowires with the similar weight percent of Pd (red dash) and Au (blue straight) nanoparticle composited at the current density of 0.4 A g−1c. Further improvement was observed with 3 wt% addition of Pd nanoparticles (red straight) onto bio MO nanowires. (d) The specific capacities of MO nanoparticles (orange), bio MO nanowires (blue), bio MO nanowires with PAA wrapping (dark yellow), Pd/bio MO nanowires (red) electrodes including s.d. error bars (154~854 mAh g−1c). Each sample type was made and tested at least triplicate. (e) The first cycling voltage profile of Li-O2batteries with the fixed discharge capacity of 4,000 mAh g−1c(400 mAh g−1c+catalyst) for MO nanoparticles (blue), bio MO nanowires (dark yellow) and Pd/bio MO nanowires (red) at the current density of 1 A g−1c. Each electrode was composed of 8 wt% of carbon and was cycled in 2–4.15 V voltage windows. (f) The cycling performance of Li-O2battery electrodes composed of MO nanoparticles (blue), bio MO nanowires (dark yellow) and Pd/bio MO nanowires (red) at the current density of 1 A g−1c(0.1 A g−1c+catalyst) with the two different fixed discharge capacities of 2,000 and 4,000 mAh g−1c(200, 400 mAh g−1c+catalyst). The circular shape indicates discharge capacities (for 2,000 and 4,000 mAh g−1c), the triangle indicates charge capacities (until 4.15 V) for 2,000 mAh g−1cand the inverted triangle indicates charge capacities for 4,000 mAh g−1c. Each electrode was composed of 8 wt% carbon. All of electrochemical tests reported in this work were repeated for at least six different devices. Figure 3: The electrochemical performance of Li-O 2 batteries. ( a ) The first galvanostatic cycle of MO nanoparticles (blue) and bio MO nanowires (red) at a current density of 0.4 A g −1 c (~0.044 mA cm −2 ) with 0.1 M LiClO 4 /DME electrolytes under 1 atm oxygen. ( b ) XRD patterns of bio MO nanowire electrodes at the pristine state (blue), the end of the first full discharge until 2.2 V (dark yellow) and the end of the first full charge until 4.15 V (red) under 0.4 A g −1 c of current density. ( c ) The first galvanostatic cycle of bio MO nanowires with the similar weight percent of Pd (red dash) and Au (blue straight) nanoparticle composited at the current density of 0.4 A g −1 c . Further improvement was observed with 3 wt% addition of Pd nanoparticles (red straight) onto bio MO nanowires. ( d ) The specific capacities of MO nanoparticles (orange), bio MO nanowires (blue), bio MO nanowires with PAA wrapping (dark yellow), Pd/bio MO nanowires (red) electrodes including s.d. error bars (154~854 mAh g −1 c ). Each sample type was made and tested at least triplicate. ( e ) The first cycling voltage profile of Li-O 2 batteries with the fixed discharge capacity of 4,000 mAh g −1 c (400 mAh g −1 c+catalyst ) for MO nanoparticles (blue), bio MO nanowires (dark yellow) and Pd/bio MO nanowires (red) at the current density of 1 A g −1 c . Each electrode was composed of 8 wt% of carbon and was cycled in 2–4.15 V voltage windows. ( f ) The cycling performance of Li-O 2 battery electrodes composed of MO nanoparticles (blue), bio MO nanowires (dark yellow) and Pd/bio MO nanowires (red) at the current density of 1 A g −1 c (0.1 A g −1 c+catalyst ) with the two different fixed discharge capacities of 2,000 and 4,000 mAh g −1 c (200, 400 mAh g −1 c+catalyst ). The circular shape indicates discharge capacities (for 2,000 and 4,000 mAh g −1 c ), the triangle indicates charge capacities (until 4.15 V) for 2,000 mAh g −1 c and the inverted triangle indicates charge capacities for 4,000 mAh g −1 c . Each electrode was composed of 8 wt% carbon. All of electrochemical tests reported in this work were repeated for at least six different devices. Full size image The major discharge product obtained after the first discharge of bio MO nanowire electrodes was Li 2 O 2 confirmed by XRD in Fig. 3b . The XRD data of discharged electrode match well to the reference XRD pattern of Li 2 O 2 (orange star, powder diffraction file number 01-074-0115). There was no other major discharge product observed except Li 2 O 2 . In previous reports, MOs have been shown to produce a LiOH phase during the discharge [38] , [49] because of the structural water or hydroxyl residues. The Li-O 2 battery performance of dehydrated (thermal treatments at 160 °C for 2 h) bio MO nanowires was investigated to eliminate any possible contributions from water molecules or hydroxyl groups. The thermally treated nanowires showed a similar discharge capacity of 9,206 mAh g −1 c at 0.4 A g −1 c ( Supplementary Fig. S7 , blue) compared with nanowires without heat treatments, although structural water decreased from 3.2 to 1.5 wt% of electrodes after heat treatment ( Supplementary Fig. S6 ). Thus, the LiOH formation is negligible in this Li-O 2 battery performance. Battery performances of Pd/Au-loaded bio MO nanowires The hybrid nanostructure composed of Pd nanoparticles and bio MO nanowires exhibited improvement of the Li-O 2 battery discharge capacity. The first galvanostatic cycle of Au/bio MO nanowires and Pd/bio MO nanowires were compared with approximately the same amount of Au (1.7 wt%) and Pd (1.1 wt%) incorporations in each nanocomposited electrode. After the addition of only ~1 wt% of Au or Pd nanoparticles, the first discharge capacities of Au/bio MO nanowires and Pd/bio MO nanowires (cutoff voltage at 2.2 V versus Li/Li + ) were improved by 8% (Au) and 15.5% (Pd) compared with bare bio MO nanowires (at 0.4 A g −1 c , Fig. 3c , Au: blue straight, Pd: red dashed). In addition, the Pd/bio MO nanowire electrodes showed ~60 mV higher discharge voltage than Au/bio MO nanowires as can be observed from Fig. 3c . The higher discharge voltage of Pd/bio MO nanowires than Au/bio MO nanowires in the first galvanostatic cycle of Li-O 2 electrodes may be attributed to the attractive interaction between Pd and oxygen [52] . Moreover, although Pd has a lower contrast than Au on TEM observation because of its lower atomic mass, large (greater than 5 nm) Pd nanoparticles on bio MO nanowires were rarely observed than Au nanoparticles-decorated bio MO nanowires ( Supplementary Fig. S5 ); hence, the smaller nanoparticle distribution of Pd/bio MO nanowires in a given synthetic conditions may improve the battery performances. Thus, the surface electrocatalytic functionality of bio MO nanowires was easily tuned by the composite synthesis method developed here. The capability to store lithium peroxide was further improved by increasing Pd incorporations from 1.1 to 3 wt% of Pd/bio MO nanowires electrodes. With 3 wt% of Pd incorporation, a 45% improvement of the first specific capacity of bio MO nanowires ( Fig. 3c , red straight, 13,347 mAh g −1 c , 1,008 mAh g −1 c+catalyst+Li2O2 ) was achieved at 0.4 A g −1 c . This is the highest specific capacity under a high applied current (0.4 A g −1 c and 0.22 A g −1 c+catalyst ) among all manganese oxide-based electrodes reported to date [38] , [53] . The formation of Li 2 O 2 after discharge and its decomposition during the charge (oxygen evolution was detected by gas chromatography in Supplementary Table S1 ) with Pd/bio MO nanowire electrodes was also confirmed by Raman spectroscopy in Supplementary Fig. S8 . No significant amount of side product (for example, Li 2 CO 3 ) can be detected by XRD and Raman, suggesting that DME is largely stable during discharge [54] . We believe the enhanced discharge capacity of Pd/bio MO nanowires originated from the better utilization of porous electrode spaces by improving the electrochemical active surface area and surface conductivity of bio MO nanowires. The Pd nanoparticles located on the surface of the bio MO nanowires facilitated ORR reactions and improved the electronic conduction throughout the Li 2 O 2 layers allowing further discharge product depositions. The differences in the charging profile of the 3 wt% Pd-MO nanowires compared with the bare bio MO nanowires ( Fig. 3a ) can be associated with the increased thickness of Li 2 O 2 layer of the 3 wt% Pd/bio MO nanowires (~4 nm Li 2 O 2 ) compared with the bare bio MO nanowires (~2.6 nm Li 2 O 2 ) because of larger discharge capacity. However, the charging potential of Pd/bio MO nanowires after decomposing 0.05 μAh cm −2 true of Li 2 O 2 was still ~100 mV lower than that of catalyst-free, carbon electrode [55] at the same depth of discharge, ~1 μAh cm −2 true (the true electrode surface area-specific capacities; the detail calculation method is included in the Methods section). This lower OER potential compared with catalyst-free electrodes suggests the catalytic function of Pd/bio MO nanowires even after the deep discharge in Li-O 2 battery. The following (second) cycle profile of MO nanoparticles, bio MO nanowires, Au (1.7 wt%)/bio MO nanowires, Pd (1.1 wt%)/bio MO nanowires and Pd (3 wt%)/bio MO nanowires are included in Supplementary Fig. S9 and Supplementary Table S2 . The second charging profile showed enhanced performance over previous manganese oxides-based electrode at ~6 times higher current density [38] , and further studies to improve the cycle life after the deep discharge remains as future work. To clarify the role of Pd nanoparticles, PAA-wrapped bio MO nanowires were tested as Li-O 2 battery electrodes under the same test conditions. The first discharge capacity of the PAA/bio MO nanowires electrode was 9,722 mAh g −1 c ( Supplementary Fig. S7 , green), which is only a 5% improvement of bio MO nanowire electrodes. This small improvement of discharge capacity could be attributed to the decreased aggregation between bio MO nanowires after PAA stabilization. The average value of discharge capacity can be seen in Fig. 3d . Therefore, the increased first discharge capacity of Pd/bio MO nanowire composites originated from Pd nanoparticle incorporation onto bio MO nanowires, not from the PAA wrapping. We expect that this methodology can be easily applied to other promising ORR or OER candidate materials to develop efficient catalyst structures for Li-O 2 batteries in future studies. Lowered carbon mass in cycling electrodes The catalyst nanostructure designed in this work, Pd/bio MO nanowires, allowed for an electrode with greatly decreased carbon content (8 wt%) in the catalyst electrodes to improve cycle life of Li-O 2 battery. Although carbon functions as a conducting agent and an ORR catalyst, it can also reduce the cycle life because side products can be formed at the carbon/electrolyte or carbon/Li 2 O 2 interface in electrodes with ether-based electrolytes [56] . By reducing carbon amounts in our electrodes, cycle life of Li-O 2 batteries was enhanced at high-current densities (1 A g −1 c , 0.1 A g −1 c+catalyst ) even under relatively low charging cutoff voltage (4.15 V). The cycling tests were conducted by limiting the discharge capacity to 2,000 mAh g −1 c (200 mAh g −1 c+catalyst ) or 4,000 mAh g −1 c (400 mAh g −1 c+catalyst , 299 mAh g −1 c+catalyst+Li2O2 ) following the previous works method [3] , [10] . Similar to the first discharge-specific capacity, the cycle life of Li-O 2 batteries was gradually enhanced as the catalyst structure changed from MO nanoparticles to nanowires and finally to composite Pd/bio MO nanowires ( Fig. 3e,f , Supplementary Figs S10–12 ). In particular, the OER overpotential was lowered as the surface area of catalyst electrodes as well as the surface conductivity of bio MO nanowires was improved by Pd incorporation ( Fig. 3e ) after being discharged to 4,000 mAh g −1 c (400 mAh g −1 c+catalyst ). Thus, the first cycling round trip efficiencies of MO nanoparticles, bio MO nanowires and Pd/bio MO nanowires was improved from 75%, 77.7 to 79.2%, respectively, as the cathode was rationally designed. The aggregated microstructure of MO nanoparticles limited the Li-O 2 battery cycle life to 10 cycles with 4,000 mAh g −1 c (299 mAh g −1 c+catalyst+Li2O2 ) at 1 A g −1 c (0.1 A g −1 c+catalyst ). The bio MO nanowires showed cycle retentions up to 20 cycles because of the high porosity and large catalytic surface area of the electrodes. After incorporating Pd nanoparticles, the discharge capacity of Li-O 2 batteries maintained stable to 50 cycles ( Fig. 3f , Supplementary Fig. S10 ). When the depth of discharge capacity was fixed to 2,000 mAh g −1 c (at 1 A g −1 c , 0.1 A g −1 c+catalyst ), these electrodes showed a longer cycle life with a similar cycling performance trend. Each MO nanoparticles, bio MO nanowires and Pd/bio MO maintained the 2,000 mAh g −1 c of discharge capacity up to 22, 47 and 58 cycles, respectively ( Fig. 3f , Supplementary Fig. S11 ). The reversible cycling number with Pd/bio MO nanowire electrodes is smaller than the recently reported [3] , [47] , which might be because of the instability of electrolyte or the reactivity between carbon and oxygen reduction intermediates [56] , [57] . This can be observed from the charging cycle profile in Supplementary Figs S10–12 , resulting in the faster decay of charging capacity than the discharging capacity, as cycling number increased in Fig. 3f . Ongoing and future work will be focused on developing stable electrolytes and carbon-free electrodes to enhance the cycling of these electrodes. To investigate the effect of carbon on cycling of Li-O 2 batteries, electrodes were prepared with 44 wt% of carbon. The cycle life of bio MO nanowires and Pd/bio MO nanowires decayed faster than those of low-carbon electrodes under the same fixed discharge capacity (728 mAh g −1 c , 400 mAh g −1 c+catalyst ) and current density (1 A g −1 c , 0.1 A g −1 c+catalyst ). The observed cycle number was 17, 21 and 30 for MO nanoparticles, bio MO nanowires and Pd/bio MO nanowires, respectively ( Supplementary Fig. S12 ). Although the electronic conductivity was higher for 44 versus 8 wt% carbon electrodes, side products can be formed in the high-carbon electrodes during cycling [56] counteracting the kinetic advantage in Li-O 2 battery performance. Therefore, we believe that Pd/bio MO nanowires are a viable material platform for long-lasting, high-capacity Li-O 2 batteries. Using a biological template, a new catalyst electrode was developed that increased capacity (13,350 mAh g −1 c ; 7,340 mAh g −1 c+catalyst at 0.4 A g −1 c ) and cycle life (50 cycles with 4,000 mAh g −1 c ; 400 mAh g −1 c+catalyst at 1 A g −1 c ; 0.4 A g −1 c+catalyst ) of Li-O 2 batteries at the highest gravimetric current density compared with other transition metal oxide-based electrodes in literatures [10] , [38] . These templates allowed the formation of high aspect ratio manganese oxide nanowires wrapped in 3 wt% Pd nanoparticles facilitating compositional control that outperforms materials made by mechanical mixing [58] . These high aspect ratio bio MO nanowires formed a porous network that maximizes the interaction between the catalyst and the discharge products (Li 2 O 2 ) thus increasing reversibility and generating a stable cycle life of Li-O 2 batteries. Further, the Pd/bio MO nanowires allowed the implementation of low-carbon electrode batteries improving battery cycle life. We believe that this template is readily adaptable for other material combinations and can provide a platform to test various catalytic electrode materials for Li-O 2 batteries and other catalytic systems. In addition, the application of biomaterials will broaden the material selection scope into diverse areas in designing Li-O 2 battery electrodes thus contributing to the development of energy storage systems. Material synthesis Manganese sulphate monohydrate (MnSO 4 ·H 2 O; Sigma-Aldrich, 2.4 ml of 50 mM) and sodium sulfate (Na 2 SO 4 ; Sigma-Aldrich, 2.4 ml of 50 mM) solutions were added together into 50 ml of deionized (DI) water. FC#2 viruses (1.63 × 10 13 ) were added into this solution and stirred at room temperature overnight. After the overnight incubation, potassium permanganate (KMnO 4 ; Alfa Aesar, 16 ml of 10 mM) solution was added and stirred at room temperature overnight. The final products were washed with DI water by centrifugation and collected after lyophilization. To incorporate the noble metal nanoparticles (Pd and Au), the bio MO solution was dialyzed against DI water overnight and diluted with DI water to make a final solution volume of 200 ml. PAA (M w : 2,000 g mol −1 , 0.6 g in 20 ml of DI water) was added and stirred overnight. The PAA-wrapped bio MO nanowires were collected by centrifugation and dispersed again with 240 ml of DI water. Au/Pd precursor solutions were added into the previous solution (for Au: gold (III) chloride trihydrate, HAuCl 4 ·3H 2 O, 2.17 ml of 25.4 mM for 1.7 wt% of Au in the final Au/bio MO nanowire composite electrodes. For Pd: sodium tetrachloropalladate (II), Na 2 PdCl 4 , Sigma-Aldrich, 0.612 ml of 34 mM for 3 wt% (0.408 ml of 34 mM for 1.1 wt%) of Pd in the final Pd/bio MO nanowire composite electrodes) and stirred overnight at room temperature. To reduce the metal ion, 3 ml of ethylene glycol was added to each Au/bio MO nanowire and Pd/bio MO nanowire solution for 24 h inside a brown bottle because of light sensitivity. The solution was washed three times by centrifugation with DI water and lyophilized. Material characterizations For SEM images, FEG-SEM 6700F (JEOL) was used under 5 kV with 5.9 mm of working distance (or 0.5 kV with 3 mm of WD) after coating the sample with Pd. HRTEM images were obtained with 2100, 2010 FEG (JEOL) under an accelerating voltage of 200 kV. The sample was loaded on formvar/carbon or quantifoil grids (Electron Microscopy Sciences). XRD (PANanalytical Multipurpose Diffractometer, Cu Kα radiation) patterns were collected with 0.18° per minute scan speeds under the following settings: 2° of anti-scatter slit, 6 mm of irradiated length of automatic mode and 0.04 rad of soller slit. The discharged/charged samples were collected after disassembling batteries inside an Ar-filled glove box and were covered by Kapton tape to prevent any air contamination. ICP-AES (Horiba Jobin Yvon ACTIVA-S) was used to determine the atomic ratio between manganese, gold, palladium ions of Au/bio MO nanowires and Pd/bio MO nanowires. The sample was dissolved in nitric acid (ACS reagent grade, 70%) at 50 °C overnight and diluted with DI water (Mediatech, Inc. meets WFI quality standards) to make the final nitric-acid concentration of 2% v/v for ICP-AES measurements. XPS (Physical Electronics Versaprobe II) was measured with the monochromatic Al X-ray source ( K α , 1486.6 eV) under the pass energy of 23.5 eV and the step size of 0.1 eV. The acquired XPS spectra were calibrated with adventitious carbon peak (1s) as a reference positioned at 284.8 eV. To quantify the PAA mass of the metal nanoparticles/bio MO nanowires composites, TGA (Q50 TA instrument) was used with 10 °C min −1 increasing temperature rate under nitrogen. Chemical titration for Mn oxidation state determination The average oxidation state of MO was determined by two separate chemical titration steps reported in the literature [43] . The colour change indicator (sodium diphenylamine-4-sulphonate, C 12 H 10 NNaO 3 S, Alfa Aesar) was further added during the titration. MO nanoparticles were used for titrations because the manganese oxidation state is expected to be similar to bio MO nanowires from XPS analysis and the protein residue of bio MO nanowires would cause significant errors during the titration. Electrochemical tests The lyophilized catalyst materials were further dried in a vacuum oven at 90 °C overnight before electrode preparations. The Li-O 2 electrodes were composed of Ketjan black (EC600JD, AkzoNobel), catalyst materials, LiTHion dispersion (Ion Power, USA) with the mass ratio of 44: 36: 20 for high-carbon-containing (44 wt%) electrodes and the mass ratio of 8: 72: 20 for low-carbon-containing (8 wt%) electrodes. These three components were dissolved into 2-propanol and mixed overnight using a bath sonicator to get homogeneous slurry mixtures. The mixture was spread on the separator (Celgard, PP2075) by tape casting methods and dried in a vacuum oven at 80 °C for 2 h. The dried slurry was punched into circle electrodes with diameters of 1.27 cm, and the mass of each electrode was measured (0.1–0.3 mg cm −2 ) following further drying in vacuum oven at 80 °C overnight before the electrochemical test. Inside the Ar-filled glove box, the catalyst electrode was soaked with the electrolyte in advance (0.1 M LiClO 4 in DME, Novolyte) and assembled into the Li-O 2 battery cell designed by our lab. Metallic Li foils (negative electrode), two layers of separators, catalyst electrodes and a positive electrode current collector (316 stainless steel mesh) were sequentially put on the cell and additional electrolyte (100 μl) was added. After the assembly, the Li-O 2 battery cell was purged with oxygen (Airgas, Ultra Pure Carrier grade) and closed at 1.08 atm. The purged cell was allowed to rest at least 2 h before the electrochemical test. The first cycle of Li-O 2 battery cell was tested by galvanostatic measurements at 0.4 A g −1 c with a Solartron Analytical 1470E potentiostat. For the cycling tests, the pressure of the Li-O 2 battery cell was adjusted again to 1.08 atm after 16 cycles and 1 A g −1 c of current was applied. The Li-O 2 battery performance with different electrolytes The first galvanostatic cycle of bio MO nanowires was tested with 1 M lithium triflate (LiCF 3 SO 3 ) in tetra(ethylene)glycol dimethyl ether (TEGDME) to investigate the Li-O 2 performance dependence on electrolytes. Here bio MO nanowire electrodes with LiCF 3 SO 3 /TEGDME exhibited higher charging overpotential as well as lower first discharge capacity ( Supplementary Fig. S7 , red, 8,766 mAh g −1 c at 0.4 A g −1 c ). Further, the coulombic efficiency of nanowire electrodes dropped from 92.6% (0.1 M LiClO 4 in DME) to 61.5% (1 M LiCF 3 SO 3 in TEGDME) at the same charging cutoff voltage, 4.15 V. As increasing the test voltage windows higher than 4.15 V may evoke the electrolyte decomposition, DME was suitable for bio MO nanowire electrodes to achieve higher coulombic efficiency in lower voltage ranges. The true electrode surface area-specific capacity Here we make estimation in calculating the thickness of the discharge product, Li 2 O 2 . It is assumed that Li 2 O 2 is formed as films throughout the overall catalyst electrode with the volumetric capacity, 2698.6 mAh cm −3 . First, the true electrode surface area was calculated. The BET surface area of bio MO nanowires is 271.7 m 2 g −1 and the reported BET surface area of Ketjan black (EC600JD, AkzoNobel) is 1,400 m 2 g −1 . Thus, the true surface area can be obtained by considering the weight percentage (catalyst: Ketjan black=36: 44) of each component in electrode, resulting in 271.7 m 2 g −1 × 0.36+1,400 m 2 g −1 × 0.44=713.8 m true 2 g −1 c+catalyst . As 13,347 mAh g −1 c corresponds to 7,340.8 mAh g −1 c+catalyst , the true electrode surface area-specific capacity is ≈1.0 μAh cm −2 true . How to cite this article: Oh, D. et al. Biologically enhanced cathode design for improved capacity and cycle life for lithium-oxygen batteries. Nat. Commun. 4:2756 doi: 10.1038/ncomms3756 (2013).